Designing high-performance layered thermoelectric materials through orbital engineering Thermoelectric technology, which possesses potential application in recycling industrial waste heat as energy, calls for novel high-performance materials. The systematic exploration of novel thermoelectric materials with excellent electronic transport properties is severely hindered by limited insight into the underlying bonding orbitals of atomic structures. Here we propose a simple yet successful strategy to discover and design high-performance layered thermoelectric materials through minimizing the crystal field splitting energy of orbitals to realize high orbital degeneracy. The approach naturally leads to design maps for optimizing the thermoelectric power factor through forming solid solutions and biaxial strain. Using this approach, we predict a series of potential thermoelectric candidates from layered CaAl 2 Si 2 -type Zintl compounds. Several of them contain nontoxic, low-cost and earth-abundant elements. Moreover, the approach can be extended to several other non-cubic materials, thereby substantially accelerating the screening and design of new thermoelectric materials. With the gradual depletion of fossil fuels and the growing pressure of the global warming, developing reliable and sustainable approaches for energy conversion is a key challenge for our society. Thermoelectric (TE) devices, which can directly and reversibly convert heat into electricity, have potential applications in waste-heat recovery, air conditioning and refrigeration [1] , [2] . However, the application of TE devices is critically limited by their low efficiencies, which are determined by the performance of the materials. Numerous efforts worldwide thus focus on optimizing current TE materials and developing novel TE materials with enhanced performance [3] , [4] , [5] , [6] , [7] , [8] , [9] . The performance of TE materials is governed by the dimensionless figure of merit, zT=α 2 σT/κ , where α is the Seebeck coefficient, σ is the electrical conductivity, κ is the thermal conductivity and T is the absolute temperature. Accordingly, enhanced zT value requires a combination of excellent electrical transport properties, quantified by the TE power factor PF =α 2 σ , and low thermal conductivity. Several successful concepts, including nano-structuring [10] and the inclusion of loosely bound rattlers [11] , have been developed to systematically reduce the lattice thermal conductivity. On the other hand, a systematic optimization of the electronic properties, which often exhibit a highly nontrivial dependence on atomic structure, still poses a big challenge. High-throughput computational screening allows the identification of compounds with high power factors via electronic transport calculations [12] , [13] . The physical insight from the approach is, however, mainly limited to the rationalization of the calculated properties. Furthermore, derived compounds, for example, a high-performing alloy of two low-performing compounds, can be overlooked. How alloying can optimize the PF by alignment of band edges has been demonstrated experimentally [5] , [14] , [15] and theoretically [16] , [17] . However, despite the intuitive appeal of this approach, it has only been applied to a few cubic or pseudo-cubic alloys. This might be attributed to the limited insight into the underlying bonding orbitals at the band edges, which makes it difficult to extend the approach to new materials. Here, taking layered CaAl 2 Si 2 -type Zintl compounds as an example, we combine first principles calculations and reported experimental data [18] , [19] , [20] , [21] , [22] , [23] , [24] , [25] , [26] , [27] , [28] , [29] , [30] , [31] , [32] , [33] to demonstrate how the TE properties can be rationalized in terms of a simple crystal field scheme of orbitals splitting. Thereby, a powerful selection rule only based on band structure parameters is established as a simplified descriptor of electrical transport performance. Using the screening rule, we identify a few promising TE candidates with nontoxic, inexpensive and earth-abundant elements from CaAl 2 Si 2 -type Zintl compounds. It is shown how the selection rule naturally leads to strategies for rationally optimizing the TE PF through solid solution map and biaxial strain engineering. Finally, the strategy is reasonably extended to several other types of materials including chalcopyrite, metal dichalcogenide and lithium intercalated metal dichalcogenide. The orbital engineering approach presented here thus provides insightful guidance for the search and design of novel promising TE materials with good electronic transport properties. Orbital characteristics and electronic transport properties AB 2 X 2 Zintl compounds crystallize in trigonal (space group: P m 1) CaAl 2 Si 2 -type structures, where A is an alkaline-earth or a divalent rare-earth element, B is a transition-metal or a main group element, X normally comes from group 15 and 14 (ref. 34 ). Generally, layered AB 2 X 2 Zintl compounds can be described as trigonal monolayers of A 2+ cations in the a - b plane separating [B 2 X 2 ] 2− covalently bound slabs ( Fig. 1a ) [27] . These Zintl compounds are known by the virtue of low thermal conductivity [35] . Furthermore, the wide variety of compositions covered by this type of compounds provides considerable chemical tunability of the transport properties. However, their complicated chemical bonds, described in detail in ref. 34 , make it a big challenge to systematically optimize the electronic transport properties. 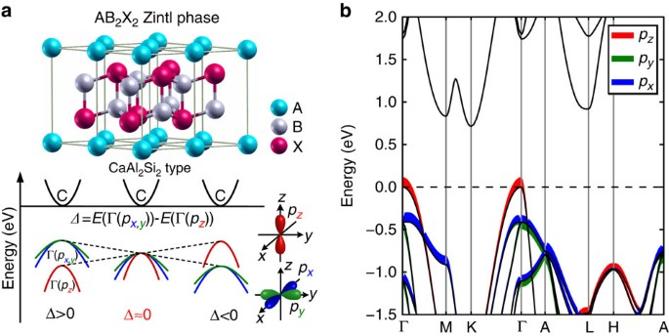Figure 1: Orbital engineering to realize threefold degenerateporbitals in layered CaAl2Si2-type Zintl compounds. (a) Crystal structure and electronic bands of CaAl2Si2-type Zintl compounds. Nondegenerate band Γ(pz) and doubly degenerate band Γ(px,y) are mainly composed ofpzandpx,yorbitals from anions, respectively.Δis the crystal field splitting energy betweenpx,yandpzorbitals at theΓpoint. (b) Orbital-projected band structure of representative CaAl2Si2-type Zintl compound Mg3Sb2with negativeΔvalue.px,pyandpzorbitals of Sb anions are projected on the band structure. Curve width indicates the relative weight of the component. Two representative compounds Mg3Sb2(Δ<0) and SrZn2Sb2(Δ>0,Supplementary Fig. 2) are used to demonstrate theporbital characteristics of CaAl2Si2-type Zintl materials. Figure 1: Orbital engineering to realize threefold degenerate p orbitals in layered CaAl 2 Si 2 -type Zintl compounds. ( a ) Crystal structure and electronic bands of CaAl 2 Si 2 -type Zintl compounds. Nondegenerate band Γ( p z ) and doubly degenerate band Γ( p x,y ) are mainly composed of p z and p x,y orbitals from anions, respectively. Δ is the crystal field splitting energy between p x,y and p z orbitals at the Γ point. ( b ) Orbital-projected band structure of representative CaAl 2 Si 2 -type Zintl compound Mg 3 Sb 2 with negative Δ value. p x , p y and p z orbitals of Sb anions are projected on the band structure. Curve width indicates the relative weight of the component. Two representative compounds Mg 3 Sb 2 ( Δ <0) and SrZn 2 Sb 2 ( Δ >0, Supplementary Fig. 2 ) are used to demonstrate the p orbital characteristics of CaAl 2 Si 2 -type Zintl materials. Full size image The basic idea of the present paper is illustrated in Fig. 1a . The AB 2 X 2 Zintl compounds are intrinsically p-doped [36] and the electronic transport properties depend sensitively on the degeneracy of the valence band edges around the Brillouin zone centre at the Γ point. The valence band edge is dominated by the p orbital characteristics of the X anions (see Fig. 1b and Supplementary Figs 1 and 2 for details). Cubic symmetry would result in threefold degenerate p orbitals at Γ point because of the equivalency of the x , y , z directions in the Brillouin zone. However, owing to the effect of the crystal field splitting (see Supplementary Note 1 for details. The effect of spin orbit coupling is discussed in Supplementary Note 2. ), the p z orbital is separated from the p x and p y orbitals in layered materials. As a result, the valence bands at the Γ point split into a doubly degenerate band Γ( p x,y ) and a nondegenerate band Γ( p z ), mainly composed, respectively, of p x,y and p z orbitals from anions ( Fig. 1 ). The energy difference between these two bands is defined as the crystal field splitting energy, namely, Δ = E (Γ( p x,y ))− E (Γ( p z )). In general, Γ( p x,y ) is a heavy hole band, whereas Γ( p z ) is a light hole band. It is desirable for optimizing electrical transport performance that Γ( p x,y ) band and Γ( p z ) band are nearly degenerate [5] , [15] , [16] . Thus, the magnitude of Δ (| Δ |) can be used to evaluate the deviation from cubic-like threefold degeneracy of p orbitals at the band edges and thereby electrical transport properties. The deviation decreases as | Δ | gets smaller, and orbital degeneracy is effectively increased when Δ value is around zero. Therefore, orbital engineering is here understood as the reconstruction of cubic-like threefold degenerate p orbitals at the band edges in layered compounds through the manipulation of the relative energies of p x , p y and p z orbitals (see Fig. 1a for details). 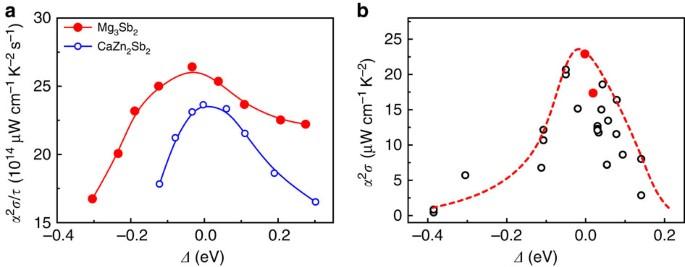Figure 2: The dependence of thermoelectric power factors on crystal field splitting energy. (a) Calculated power factorsα2σ/τat 600 K of two representative CaAl2Si2-type Zintl compounds, Mg3Sb2and CaZn2Sb2, with negative and positiveΔ, respectively. The crystal field splitting energyΔis varied by slightly tuning lattice parametersaandc.For eachΔvalue, the theoretical power factorα2σ/τis calculated at a hole concentrationp=1020cm−3. A similar dependence ofα2σ/τonΔis observed if the optimal carrier concentration is used (Supplementary Fig. 5). The solid lines represent fitted curves using aBspline.τis the constant carrier relaxation time. (b) Experimental power factors18,19,20,21,22,23,24,25,26,27,28,29,30,31,32,33α2σat 600 K as a function of the crystal field splitting energyΔin CaAl2Si2-type Zintl compounds. Solid solutions YbCd1.6Zn0.4Sb2and EuZn1.8Cd0.2Sb2withzTvalues18,19above unity are marked in red. Experimental reported Zintl compounds18,19,20,21,22,23,24,25,26,27,28,29,30,31,32,33studied here include YbCd2Sb2, YbZn2Sb2, EuZn2Sb2, EuCd2Sb2, CaZn2Sb2, SrZn2Sb2, CaMg2Bi2, YbMg2Bi2, Mg3Bi2, Mg3Sb2, Eu(Zn1−xCdx)2Sb2(x=0.1, 0.3 and 0.5), Yb(Zn1−xCdx)2Sb2(x=0.5 and 0.8) and Yb1−xEuxCd2Sb2(x=0.25). The curve is guide to the eye, showing the best values corresponding to optimum carrier concentrations. The data points include varying carrier concentrations for the same compound reported in different references. Materials with carrier concentrations deviating from optimal values are below the curve. Figure 2a shows the calculated dependence of the PF on Δ for two representative CaAl 2 Si 2 -type Zintl compounds Mg 3 Sb 2 and CaZn 2 Sb 2 with, respectively, negative and positive Δ values (see also Supplementary Figs 3a, 4 and 5 for details). The theoretical power factors increase with the increasing Δ value and then decrease, showing peak values when Δ approaches zero, which is consistent with the above discussion. Figure 2b (see also Supplementary Fig. 3b for details ) shows the experimental power factors of all reported TE Zintl compounds [18] , [19] , [20] , [21] , [22] , [23] , [24] , [25] , [26] , [27] , [28] , [29] , [30] , [31] , [32] , [33] with the CaAl 2 Si 2 -type structure and their correlation with the calculated Δ . The result confirms that the peak power factors are obtained as Δ ≈ 0, fully consistent with the trend of theoretical power factors. Moreover, the tendency of the experimental zT values at different temperatures shown in Fig. 3 and Supplementary Fig. 6 strongly resembles the dependence of the power factors on Δ . Considerably enhanced zT values are observed when Δ is around zero. In a few reported CaAl 2 Si 2 -type Zintl compounds with nearly zero Δ values, the optimum zT values [18] , [19] of 1.0–1.2 are achieved at the temperature range of 600–700 K. Figure 2: The dependence of thermoelectric power factors on crystal field splitting energy. ( a ) Calculated power factors α 2 σ/τ at 600 K of two representative CaAl 2 Si 2 -type Zintl compounds, Mg 3 Sb 2 and CaZn 2 Sb 2 , with negative and positive Δ , respectively. The crystal field splitting energy Δ is varied by slightly tuning lattice parameters a and c. For each Δ value, the theoretical power factor α 2 σ/τ is calculated at a hole concentration p =10 20 cm −3 . A similar dependence of α 2 σ/τ on Δ is observed if the optimal carrier concentration is used ( Supplementary Fig. 5 ). The solid lines represent fitted curves using a B spline. τ is the constant carrier relaxation time. ( b ) Experimental power factors [18] , [19] , [20] , [21] , [22] , [23] , [24] , [25] , [26] , [27] , [28] , [29] , [30] , [31] , [32] , [33] α 2 σ at 600 K as a function of the crystal field splitting energy Δ in CaAl 2 Si 2 -type Zintl compounds. Solid solutions YbCd 1.6 Zn 0.4 Sb 2 and EuZn 1.8 Cd 0.2 Sb 2 with zT values [18] , [19] above unity are marked in red. Experimental reported Zintl compounds [18] , [19] , [20] , [21] , [22] , [23] , [24] , [25] , [26] , [27] , [28] , [29] , [30] , [31] , [32] , [33] studied here include YbCd 2 Sb 2 , YbZn 2 Sb 2 , EuZn 2 Sb 2 , EuCd 2 Sb 2 , CaZn 2 Sb 2 , SrZn 2 Sb 2 , CaMg 2 Bi 2 , YbMg 2 Bi 2 , Mg 3 Bi 2 , Mg 3 Sb 2 , Eu(Zn 1− x Cd x ) 2 Sb 2 ( x =0.1, 0.3 and 0.5), Yb(Zn 1− x Cd x ) 2 Sb 2 ( x =0.5 and 0.8) and Yb 1− x Eu x Cd 2 Sb 2 ( x =0.25). The curve is guide to the eye, showing the best values corresponding to optimum carrier concentrations. The data points include varying carrier concentrations for the same compound reported in different references. Materials with carrier concentrations deviating from optimal values are below the curve. 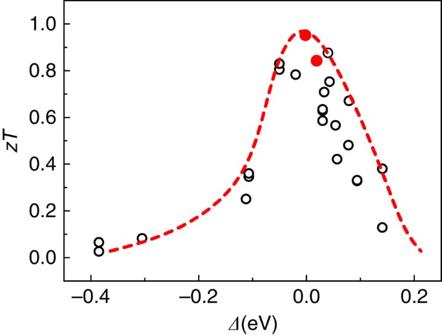Figure 3:zTvalues at 600 K versus calculatedΔvalues in CaAl2Si2-type Zintl compounds. ExperimentalzTvalues are collected from refs18,19,20,21,22,23,24,25,26,27,28,29,30,31,32,33. YbCd1.6Zn0.4Sb2and EuZn1.8Cd0.2Sb2solid solutions withzTvalues18,19above unity at high temperature are marked in red. The curve is guide to the eye, showing the maximum values corresponding to optimal carrier concentrations. Full size image Figure 3: zT values at 600 K versus calculated Δ values in CaAl 2 Si 2 -type Zintl compounds. Experimental zT values are collected from refs 18 , 19 , 20 , 21 , 22 , 23 , 24 , 25 , 26 , 27 , 28 , 29 , 30 , 31 , 32 , 33 . YbCd 1.6 Zn 0.4 Sb 2 and EuZn 1.8 Cd 0.2 Sb 2 solid solutions with zT values [18] , [19] above unity at high temperature are marked in red. The curve is guide to the eye, showing the maximum values corresponding to optimal carrier concentrations. Full size image Moreover, the optimal electronic transport performance of TE materials is proportional to the weighted mobility, μ 0 ( m */ m e ) 3/2 , where μ 0 is the intrinsic mobility, m * is the density-of-states effective mass and m e is the mass of an electron [2] , [5] . Using the single parabolic band model and the assumption of acoustic phonon scattering mechanism, the values of μ 0 ( m */ m e ) 3/2 and maximum zT at optimal carrier concentrations for many reported CaAl 2 Si 2 -type Zintl compounds [18] , [20] , [21] , [22] , [23] , [25] , [26] , [27] , [28] , [31] , [32] , [33] , [37] are calculated from published Hall data ( Supplementary Table 1 ). The correlation between μ 0 ( m */ m e ) 3/2 (optimum zT ) and Δ is demonstrated in Supplementary Fig. 7 . As expected, μ 0 ( m */ m e ) 3/2 (optimum zT ) also undergoes a peak value when Δ is around zero. Screening rule for high electrical transport performance Based on the established relationships between power factor, figure of merit ( zT ), orbital degeneracy and Δ , we are able to define a selection rule, that is, maintaining the crystal field splitting energy around zero (zero- Δ rule) to obtain good electrical transport performance and thereby high TE performance. Many CaAl 2 Si 2 -type Zintl compounds and corresponding Δ values are listed in Supplementary Table 2 . Combining the selection criterion −0.06≤ Δ ≤0.06 and band gap E g <1.5 eV, we start the search for promising TE candidates from Zintl compounds. Besides those that have been confirmed by previous references [18] , [19] , [20] , [21] , [22] , [23] , [24] , [25] , [26] , [27] , [28] , [29] , [30] , [31] , [32] , [33] , compounds such as SrMg 2 Sb 2 , BaMg 2 Sb 2 , SrMg 2 Bi 2 and BaMg 2 Bi 2 are expected to show good electronic transport properties as well as TE performance. It is worthwhile to note that among these compounds potential TE candidates SrMg 2 Sb 2 and BaMg 2 Sb 2 contain earth-abundant, nontoxic and inexpensive elements. The screening of a large number of CaAl 2 Si 2 -type Zintl compounds shows that only a few of the Zintl compounds possess nearly zero Δ values and suitable band gaps. It is therefore crucial to develop feasible and effective approaches to manipulate crystal field splitting energy for materials design and optimization. The splitting energy between the in-plane p x,y and out-of-plane p z orbitals at the valence band maximum is mainly determined by their hybridizations. Usually, compared with p x,y orbitals, the energy level of p z orbitals at the band edge will be more sensitive to their interlayer hybridization. Thus, tuning the interlayer distance could effectively manipulate the energy level of p z orbitals and thereby crystal field splitting energy. Continuous change of the interlayer distance can be introduced by crystal deformation, which can be induced by both internally and externally applied forces. Internal forces involve chemical doping or forming solid solutions, whereas external forces include physical pressure, strain effect and so on. Here two powerful approaches, solid solution map and biaxial strain engineering, are developed to realize the tunability of Δ , which will be discussed below. 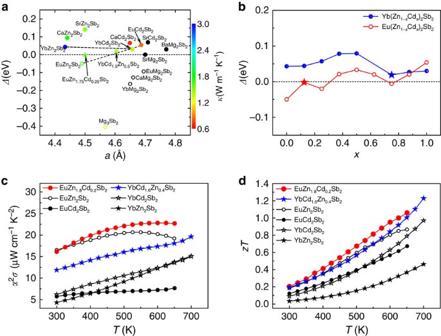Figure 4: Solid solution map for designing high-performance multinary compounds with CaAl2Si2-type structure. (a) CalculatedΔas a function of the lattice constantain CaAl2Si2-type Zintl compounds withEg<1.5 eV. The stars correspond to solid solutions YbCd1.5Zn0.5Sb2and EuZn1.75Cd0.25Sb2with nearly zeroΔvalues. Reported values18,19,20,21,22,23,24,25,26,27,28,29,30,31,32,33of thermal conductivity at 500 K are shown in colour bar. (b) CalculatedΔversus the fractionxin two representative solid solutions Yb(Zn1–xCdx)2Sb2and Eu(Zn1–xCdx)2Sb2. The stars represent solid solutions YbCd1.5Zn0.5Sb2and EuZn1.75Cd0.25Sb2with nearly zeroΔvalues. (c,d) Temperature dependence of power factors18,19α2σ(c) andzTvalues18,19(d) of YbZn2Sb2(EuZn2Sb2), YbCd2Sb2(EuCd2Sb2) and their solid solutions YbCd1.6Zn0.4Sb2and EuZn1.8Cd0.2Sb2. Solid solution map for designing multinary TE compounds Figure 4a displays the Δ versus a compound map for CaAl 2 Si 2 -type Zintl compounds, where a is the lattice constant. The values of the thermal conductivity of reported Zintl compounds [18] , [19] , [20] , [21] , [22] , [23] , [24] , [25] , [26] , [27] , [28] , [29] , [30] , [31] , [32] , [33] at 500 K are marked in the colour bar. Only a few compounds with band gaps smaller than 1.5 eV are illustrated out of the variety of Zintl compounds with CaAl 2 Si 2 -type structure. The compound maps as a function of, respectively, lattice constant a and band gap, with nearly all CaAl 2 Si 2 -type Zintl compounds are depicted in Supplementary Fig. 8a,b . In order to achieve an ideal Δ =0 value, one can select two or more compounds with positive (larger than 0) and negative (smaller than 0) Δ values and attempt to form a solid solution or mixture with Δ ≈0 by slightly adjusting the molar ratio of the constituent compounds. This strategy constructs the overall picture of designing multinary CaAl 2 Si 2 -type Zintl compounds with ideal zero Δ values that yield good TE performance. Another possible optimizing approach is to select one compound with relatively low thermal conductivity and add it into one compound with nearly zero Δ forming a solid solution with the aim to block heat conduction without explicitly reducing the electronic transport through carefully tuning the molar ratio of the constituent compounds with poor heat conduction. Figure 4: Solid solution map for designing high-performance multinary compounds with CaAl 2 Si 2 -type structure. ( a ) Calculated Δ as a function of the lattice constant a in CaAl 2 Si 2 -type Zintl compounds with E g <1.5 eV. The stars correspond to solid solutions YbCd 1.5 Zn 0.5 Sb 2 and EuZn 1.75 Cd 0.25 Sb 2 with nearly zero Δ values. Reported values [18] , [19] , [20] , [21] , [22] , [23] , [24] , [25] , [26] , [27] , [28] , [29] , [30] , [31] , [32] , [33] of thermal conductivity at 500 K are shown in colour bar. ( b ) Calculated Δ versus the fraction x in two representative solid solutions Yb(Zn 1– x Cd x ) 2 Sb 2 and Eu(Zn 1– x Cd x ) 2 Sb 2 . The stars represent solid solutions YbCd 1.5 Zn 0.5 Sb 2 and EuZn 1.75 Cd 0.25 Sb 2 with nearly zero Δ values. ( c , d ) Temperature dependence of power factors [18] , [19] α 2 σ ( c ) and zT values [18] , [19] ( d ) of YbZn 2 Sb 2 (EuZn 2 Sb 2 ), YbCd 2 Sb 2 (EuCd 2 Sb 2 ) and their solid solutions YbCd 1.6 Zn 0.4 Sb 2 and EuZn 1.8 Cd 0.2 Sb 2 . Full size image Through density functional theory calculation, Δ values as a function of the fraction x in two selected solid solutions Yb(Zn 1− x Cd x ) 2 Sb 2 and Eu(Zn 1− x Cd x ) 2 Sb 2 are simulated and shown in Fig. 4b . The results of Yb(Zn 1− x Cd x ) 2 Sb 2 and Eu(Zn 1− x Cd x ) 2 Sb 2 prove that it is indeed feasible to realize the ideal Δ value around zero in the selected solid solutions. The calculated band structure of an exemplified solid solution EuZn 1.75 Cd 0.25 Sb 2 satisfying the nearly zero Δ value indicates that high orbital degeneracy at the valence band maxiamum is realized ( Supplementary Fig. 9 ). Both Yb(Zn 1− x Cd x ) 2 Sb 2 and Eu(Zn 1− x Cd x ) 2 Sb 2 have been studied experimentally [18] , [19] . Figure 4c,d and Supplementary Fig. 10 show the temperature dependence of power factors, zT values, and thermal conductivities of two solid solutions YbCd 1.6 Zn 0.4 Sb 2 and EuZn 1.8 Cd 0.2 Sb 2 compared with the pure ternaries. The above two solid solutions with ideal Δ values around zero exhibit greatly enhanced power factors [18] , [19] and zT values [18] , [19] compared with non-alloyed compounds, consistent with the calculations. Moreover, the thermal conductivity of YbCd 1.6 Zn 0.4 Sb 2 or EuZn 1.8 Cd 0.2 Sb 2 is comparable to one of the constituent compounds. All the above results validate that the strategy based on solid solution maps is effective in the design of complex high-performance TE materials from a range of CaAl 2 Si 2 -type Zintl compounds. According to the well-established solid solution maps, there still exists many potential solid solutions that have not been reported yet, for example, Eu 1− x Ca x Zn 2 Sb 2 , Yb 1− x Ba x Mg 2 Sb 2 , Ca(Mg 1− x Cd x ) 2 Sb 2 , Yb(Mg 1− x Zn x ) 2 Sb 2 , Ca 1− x Ba x Mg 2 Bi 2 and so on. In particular, Ca(Zn 1− x Mg x ) 2 Sb 2 , Sr 1− x Ba x Mg 2 Sb 2 and Sr(Mg 1− x Zn x ) 2 Sb 2 are promising TE candidates with earth-abundant, cheap and nontoxic chemical elements. Biaxial strain engineering to optimize zT In addition to the solid solution method, external forces like biaxial strain can also be used to manipulate the Δ value. The biaxial strain can be introduced here by the lattice mismatch between the substrate materials with selected cubic lattice and the thin film TE materials with the CaAl 2 Si 2 -type structure deposited on the substrate. The biaxial strain ɛ can be defined as ( a - a 0 )/ a 0 × 100%, where a 0 and a are the in-plane lattice parameters with unstrained and strained states, respectively. 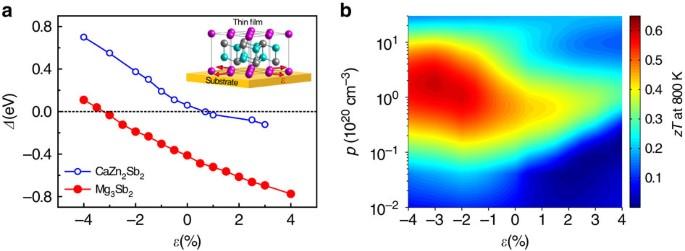Figure 5: Biaxial strain engineering to optimize TE performance of CaAl2Si2-type Zintl compounds. (a)Δversus biaxial strainɛin two representative CaAl2Si2-type Zintl compounds Mg3Sb2and CaZn2Sb2. Here biaxial strainɛis defined as (a−a0)/a0× 100%, wherea0andaare the in-plane lattice parameters with unstrained and strained states, respectively. (b) The contour map of calculatedzTvalue of Mg3Sb2at 800 K as a function of hole concentrationpand biaxial strain ɛ. Figure 5a shows Δ as a function of ɛ in two representative CaAl 2 Si 2 -type Zintl compounds, Mg 3 Sb 2 and CaZn 2 Sb 2 . As the figure depicts, a linear correlation between Δ and ɛ is observed. The value of Δ increases (decreases) linearly with the increasing magnitude of the compressive (tensile) strain. Thus, we can deduce a general optimization rule for high TE performance, that is, for Zintl compounds with positive Δ value tensile biaxial strain is more effective, whereas for Zintl compounds with negative Δ value compressive biaxial strain is preferred. According to the first-principles calculations, the calculated power factors can be continuously tuned by biaxial strain and show peak values at optimal biaxial strains corresponding to nearly zero Δ values ( Supplementary Fig. 11 ). For negative- Δ Mg 3 Sb 2 , the optimal biaxial strain turns out to be compressive, whereas for positive- Δ CaZn 2 Sb 2 , optimal biaxial strain appears to be tensile, fully consistent with the above deduction. Using semiclassical Boltzmann transport theory and experimental data [30] (see Methods for details), the dependence of zT at 800 K on carrier concentration and biaxial strain is estimated for Mg 3 Sb 2 and plotted in Fig. 5b . The maximum zT value of Mg 3 Sb 2 at 800 K at the optimal strain −3% shows around 50% enhancement compared with the value of the unstrained case. Thus, biaxial strain engineering is an effective approach for tuning and optimizing TE performance, showing potential application to thin-film materials with the CaAl 2 Si 2 -type structure. Figure 5: Biaxial strain engineering to optimize TE performance of CaAl 2 Si 2 -type Zintl compounds. ( a ) Δ versus biaxial strain ɛ in two representative CaAl 2 Si 2 -type Zintl compounds Mg 3 Sb 2 and CaZn 2 Sb 2 . Here biaxial strain ɛ is defined as ( a − a 0 )/ a 0 × 100%, where a 0 and a are the in-plane lattice parameters with unstrained and strained states, respectively. ( b ) The contour map of calculated zT value of Mg 3 Sb 2 at 800 K as a function of hole concentration p and biaxial strain ɛ. Full size image Extension of orbital engineering to several other compounds The orbital engineering approach based on zero- Δ screening rule, solid solution map and biaxial strain engineering developed here can also be used for optimizing a vast number of non-cubic compounds with similar p orbitals characteristics at the band edges. 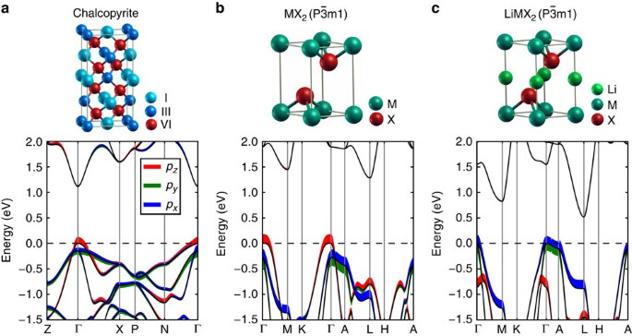Figure 6: Extension of orbital engineering to several other non-cubic compounds. (a–c) Orbital-projected band structures and crystal structures of representative chalcopyrite compound AgGaTe2(a), metal dichalcogenide ZrS2(b) and lithium intercalated metal dichalcogenide LiZrSe2(c).px,pyandpzorbitals of anions are projected on the band structures. Curve width indicates the relative weight of the component. Figure 6 and Supplementary Figure 12 show the orbital-projected band structures and density of states of AgGaTe 2 , ZrS 2 and LiZrSe 2 , which are representatives of chalcopyrites, metal dichalcogenides MX 2 (space group: P m 1) and lithium intercalated metal dichalcogenides LiMX 2 (space group: P m 1), respectively. All of these compounds possess crystal field split p orbital characteristics at the band edges, similar to the CaAl 2 Si 2 -type Zintl compounds. The results of biaxial strain engineering in chalcopyrites, metal dichalcogenides and lithium intercalated metal dichalcogenides from references (CuGaTe 2 and TiS 2 ) [38] , [39] and our own data (ZrS 2 and LiZrSe 2 ; see Supplementary Fig. 13 for details) confirm orbital engineering. Detailed information including a solid solution map of metal dichalcogenides MX 2 is provided in Supplementary Fig. 14 and Supplementary Table 3 , with the aim to guide the optimization of p -type TE performance for metal dichalcogenides. Figure 6: Extension of orbital engineering to several other non-cubic compounds. ( a – c ) Orbital-projected band structures and crystal structures of representative chalcopyrite compound AgGaTe 2 ( a ), metal dichalcogenide ZrS 2 ( b ) and lithium intercalated metal dichalcogenide LiZrSe 2 ( c ). p x , p y and p z orbitals of anions are projected on the band structures. Curve width indicates the relative weight of the component. Full size image In summary, we have proposed a novel approach to realize high orbital degeneracy at the band edges that yields good electronic transport properties and thereby high TE performance via tuning the relative energies of orbitals in layered CaAl 2 Si 2 -type Zintl compounds. We establish a simple yet insightful screening criterion: maintaining crystal field splitting energy around zero. Using the calculated Δ versus lattice parameter maps, one can conveniently choose two or more compounds to form a solid solution with the desirable zero Δ value that leads to excellent electronic transport performance. Moreover, Δ and TE performance can be continuously tuned and optimized by biaxial strain engineering. Based on the orbital engineering approach, we predict a series of potential TE candidates with CaAl 2 Si 2 -type structure. Some of them have been proved experimentally with enhanced zT values. Several predicted promising compounds contain earth-abundant, cheap and nontoxic elements. Finally, the orbital engineering strategy is rationally extended to other types of materials with the same orbital features at the band edges. Thus, we believe that orbital engineering strategy based on zero- Δ rule and augmented by solid solution map and biaxial strain engineering opens a new avenue for high-throughput computational screening of TE materials and thereby will accelerate the screening and design of new high-performance TE materials from a myriad of non-cubic compounds. Computational methods Density Functional Theory calculations were carried out using the projector-augmented wave method [40] as implemented in the Vienna ab initio simulation package [41] . HSE06 functional [42] was used to relax the internal coordinates in the unit cell, whereas the lattice parameters of CaAl 2 Si 2 -type Zintl compounds were fixed to the experimental values from the literature. Here HSE06 functional was used to get structural parameters close to the experimental values. The plane-wave energy cutoff was set at 400 eV, and a 6 × 6 × 4 Monkhorst-Pack k mesh was used for crystal structure optimization. A 12 × 12 × 8 Monkhorst-Pack k mesh and a 32 × 32 × 18 Monkhorst-Pack k mesh were used for electronic structure calculations and transport properties calculations, respectively. An energy convergence criterion of 10 −4 eV and a Hellmann-Feynman force convergence criterion of 0.008 eV Å −1 were adopted. Electronic structure calculations were implemented by combining the mBJ potential and the well-established PBE+ U method [43] , [44] , and U =4 eV (ref. 44 ) was applied on Zn 3 d states and Cd 4 d states. This method has already been successfully applied to a wide range of narrow gap semiconductors to get accurate band gaps comparable to the experimental values [43] , [44] . Electrical transport property calculations were carried out by combining the ab initio band structure calculations and the Boltzmann transport theory under the constant carrier scattering time approximation as implemented in the BoltzTraP [45] code. Calculation details of electronic structure for solid solutions, chalcopyrite (AgGaTe 2 ), metal dichalcogenides and lithium intercalated metal dichalcogenide (LiZrSe 2 ) are given in Supplementary Notes 3–5 . The calculation methods here are enough to study materials discussed in this paper ( Supplementary Fig. 15 ), but might be insufficient to be used to study strongly correlated materials such as Kondo Insulators [46] with strong hybridization of localized f electrons with electronic bands. To study the effects of biaxial strain, a variety of in-plane a lattice parameters were analysed, and for each of them, the c parameter and the atomic positions were optimized. The carrier relaxation time τ was reasonably assumed to be independent of the strain in current work as the crystal structure for each step tuned by the biaxial strain is rather small. The figure of merit zT of Mg 3 Sb 2 under biaxial strain effect ( Fig. 5b ) was calculated using the following formula: Where α , σ / τ , and κ e / τ can be directly obtained from BoltzTraP code. Thus, to obtain zT , we still need to know lattice thermal conductivity κ L and constant scattering time τ . With the lattice thermal conductivity κ L (330 K)=1.341 W m −1 K −1 of Mg 3 Sb 2 obtained from ref. 30 , κ L (800 K)=0.553 W m −1 K −1 is estimated using the reciprocal relation of κ L to T . Generally, under biaxial strain, lattice thermal conductivity is lower than that without strain because of the enhancement of phonon scattering by strain-induced defects [47] , which is beneficial to TE performance. To study the contribution to zT from electrical transport, lattice thermal conductivity here was assumed to be independent of biaxial strain. The carrier’s scattering time τ could be derived from the relation μ = eτ/m* , where μ is the carrier mobility, m* is the effective mass of carrier and e is the elementary charge. Calculation details of constant carrier scattering time τ are provided in Supplementary Note 6 and Supplementary Table 4 . How to cite this article: Zhang, J. et al. Designing high-performance layered thermoelectric materials through orbital engineering. Nat. Commun. 7:10892 doi: 10.1038/ncomms10892 (2016).